Formation of recent Pb-Ag-Au mineralization by potential sub-surface microbial activity Las Cruces is a base-metal deposit in the Iberian Pyrite Belt, one of the world’s best-known ore provinces. Here we report the occurrence of major Pb-Ag-Au mineralization resulting from recent sub-surface replacement of supergene oxyhydroxides by carbonate and sulphide minerals. This is probably the largest documented occurrence of recent microbial activity producing an ore assemblage previously unknown in supergene mineralizing environments. The presence of microbial features in the sulphides suggests that these may be the first-described natural bacteriomorphs of galena. The low δ 13 C values of the carbonate minerals indicate formation by deep anaerobic microbial processes. Sulphur isotope values of sulphides are interpreted here as reflecting microbial reduction in a system impoverished in sulphate. We suggest that biogenic activity has produced around 3.1 × 10 9 moles of reduced sulphur and 10 10 moles of CO 2 , promoting the formation of ca . 1.19 Mt of carbonates, 114,000 t of galena, 638 t of silver sulphides and 6.5 t of gold. One of the principal ecological niches for extremophilic microbes is the sub-surface environment, where there is more opportunity for the existence of anaerobic life [1] . Here, the absence of oxygen is a limiting factor for heterotrophic processes. Consequently, lithoautotrophic bacteria create microdomains with metastable mineral assemblages that are inhibited under low-temperature, oxygenated surface conditions. Recent studies suggest that nearly the same amount of biomass is present in subterranean and sub-seafloor settings as on Earth’s surface [1] , [2] , [3] , [4] . The contact between the Late Devonian–Early Carboniferous ( ca . 360–330 Ma) volcanogenic massive sulphide deposit in the Las Cruces mine (Seville, southern Spain) and unconformably overlying Cenozoic sedimentary rocks of the Guadalquivir basin ( Fig. 1a ) hosts an unusual secondary mineral assemblage that includes galena, carbonates, iron sulphides, silver-rich sulphides and gold [5] , [6] , [7] , [8] . This assemblage forms a sub-horizontal rock layer, ~3–10 m thick, which caps the tilted primary massive sulphide lens. Beneath the layer is a large secondary cementation zone, up to 40 m thick, containing abundant chalcocite that constitutes the ore currently mined at Las Cruces, making it one of the richest copper deposits worldwide (17 Mt at 6.9% Cu) [7] . At the mine, the basement-cover contact is currently the locus of a major stratiform aquifer dominated by sulphate-bearing, calcium-bicarbonate, neutral to alkaline groundwaters. 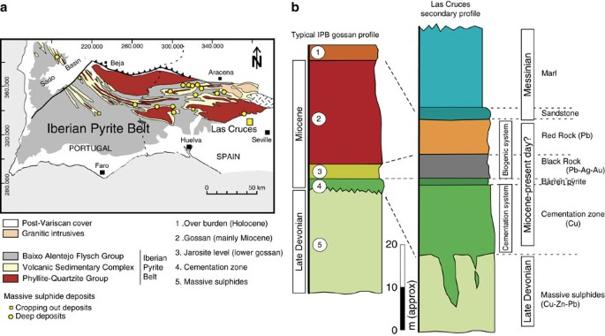Figure 1: Geologic setting of the Las Cruces mine. (a) Regional geological map showing the location of the deposit. Adapted from ref.10with permission from Elsevier; (b) idealized sections of the typical gossan of the Iberian Pyrite Belt and of the secondary mineralized zone at Las Cruces (graphical scale,ca. 20 m). Outcropping ore deposits of the Iberian Pyrite Belt have well-formed gossans. Las Cruces is an exception, with a secondary zone covered by Cenozoic sediments. The quoted ages are depositional ages for the primary massive sulphides and the sediments but are formational ages of the gossan and secondary mineralization. Figure 1: Geologic setting of the Las Cruces mine. ( a ) Regional geological map showing the location of the deposit. Adapted from ref. 10 with permission from Elsevier; ( b ) idealized sections of the typical gossan of the Iberian Pyrite Belt and of the secondary mineralized zone at Las Cruces (graphical scale, ca . 20 m). Outcropping ore deposits of the Iberian Pyrite Belt have well-formed gossans. Las Cruces is an exception, with a secondary zone covered by Cenozoic sediments. The quoted ages are depositional ages for the primary massive sulphides and the sediments but are formational ages of the gossan and secondary mineralization. Full size image The massive sulphide orebody is similar to those elsewhere in the southern part of the Iberian Pyrite Belt [9] , [10] that formed in the latest Famennian ( ca . 360 Ma) and subsequently were folded and metamorphosed during the Variscan orogeny (330–300 Ma). The Las Cruces deposit differs, however, in occurring below 150 m of Late Tortonian–Messinian ( ca . 7.2–5.3 Ma) sandstone and marl. This setting hindered its discovery and exploitation until 1994, but contributed greatly to the formation of the unusual mineral assemblages. Other massive sulphide deposits of the Iberian Pyrite Belt that were exhumed in Miocene time (<23 Ma) underwent extensive sub-aerial supergene alteration and have classical secondary alteration zones [11] . The available data suggest that some of these secondary zones formed at 7–8 Ma (ref. 11 ). Here, sulphides were weathered and the leached caps were depleted of Cu and Zn but enriched in Fe, producing the well-known orange and red gossans that overlie most of the exposed volcanogenic massive sulphide deposits of the Pyrite Belt, and that contain abundant and visually distinctive haematite and goethite. Within these deposits, the contact between the cementation zone and the gossan is the locus of a yellowish layer, several metres thick, enriched in Pb, As, Sb, Hg, Ag and Au, and having significant amounts of barite and quartz. The lead is found in cerussite, anglesite, plumbojarosite or beudantite, whereas the silver seems to occur as small amounts of argentojarosite; gold is present as sub-microscopic inclusions within the goethite [11] . At Las Cruces, this typical gossan has been replaced by a younger sulphide-carbonate assemblage, which is, to our knowledge, foreign to sub-aerial supergene environments. We interpret this unusual rock as having formed due to sub-surface metabolism of anaerobic prokaryotes under the marl unit that seals the deposit. The secondary zone In great contrast to the general behaviour of sub-aerially exposed orebodies in the Iberian Pyrite Belt and elsewhere, the gossan at Las Cruces shows a complex sequence of post-formational modifications ( Fig. 1 ). Here, the original goethite- and haematite-rich assemblage is replaced by a siderite- and galena-rich rock (Red Rock), which in turn is replaced by a younger, highly heterogeneous rock (Black Rock) having variable proportions of coarse-grained (0.5–2 mm) calcite, fine-grained (<10 μm) galena and minute acicular to globular aggregates composed of greigite and smythite. The Black Rock also contains minor amounts of intergrown acanthite, sternbergite, proustite-xanthoconite, pearceite, jamesonite, cinnabar and cassiterite; gold-rich alloys are intergrown with the carbonates and galena. Barite and quartz are common gangue minerals in both the Black and Red rocks. Thin (<1 mm) sub-vertical veins of galena penetrate through the overlying marl [12] and also cut the underlying massive sulphides. Blake [8] first suggested that both the Black and Red rocks were of bacterial origin. Bacteriomorphic structures The Black Rock contains abundant, unbranched and twisted, thread-like aggregates of galena ca . 5–10 μm in length and ≤1 μm radius located on carbonate crystals ( Fig. 2 ). These aggregates are morphologically similar to the microbial structures reported previously in the laboratory [13] and in fossil [14] , [15] geomicrobiological systems. The lack of external morphological features suggests that the galena precipitated as an extracellular polymer coating of bacteria as a result of metabolic sulphate reduction [16] . No previous records exist in natural systems of bacteriogenic structures composed of galena. Biogenic galena, to our knowledge, has only been described as a product of the bacterially mediated reduction of anglesite in discarded batteries [17] . 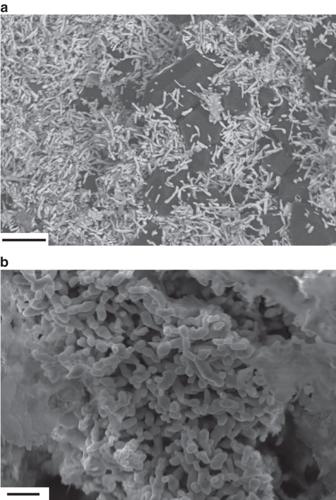Figure 2: Bacteriomorphic galena on calcite in the Black Rock. (a) Scanning electron microscope (SEM) secondary electron image (scale bar, 10 μm); (b) SEM backscattered electron image (scale bar, 5 μm). Figure 2: Bacteriomorphic galena on calcite in the Black Rock. ( a ) Scanning electron microscope (SEM) secondary electron image (scale bar, 10 μm); ( b ) SEM backscattered electron image (scale bar, 5 μm). Full size image Stable isotope geochemistry Carbon, oxygen and sulphur isotope analyses were obtained on the Red and Black rocks, as well as on the overlying marl and local groundwaters ( Table 1 ). The δ 13 C and δ 18 O values of the siderite and calcite range from −42 to −18‰ versus V-PDB (δ 13 C) and +22.1 to +27.5‰ versus V-SMOW (δ 18 O). The δ 34 S values of the sulphides (versus V-CDT) are +11.9 to +25.9‰ for galena and +16.3 to +19.5‰ for greigite–smythite. Table 1 Stable isotope composition of groundwater and carbonates and sulphides from Las Cruces. Full size table The strict localization of the Red and Black rocks in the contact zone between the paleosurface and the deformed massive sulphides, and the presence of veins of galena cutting the overlying Tertiary sediments, indicate that these rocks are not related to the in situ submarine oxidation of the massive sulphides shortly after their formation at or near the seafloor, or by much later sub-aerial processes as proposed by Knight [5] . More probably, the Red and Black rocks formed after burial beneath the Late Tortonian–Messinian sediments [8] . Both the presence of bacteria replaced by galena and the stable isotope data are consistent with replacement of the gossan being related to biogenic processes. The δ 13 C carbonate values are best interpreted as reflecting the mixing between 13 C-depleted carbon and relatively isotopically heavy carbon (δ 13 C>−9‰), with this latter end member derived from dissolved inorganic carbon (DIC; defined as ΣC (CO 2,aq +H 2 CO 3 +HCO 3 − )) in local groundwaters ( Fig. 3a and Table 1 ). The most plausible source of the isotopically light carbon is the in situ biogenic oxidation of methane and other light hydrocarbons ( Fig. 4 ); this interpretation is supported by the accumulations of light gas that are common in the Guadalquivir basin [18] . The ultimate origin of the light carbon may be thermal maturation of Palaeozoic shale within the underlying basement, a process that released gas that then ascended through fractures, accumulating below the sealing marl unit. 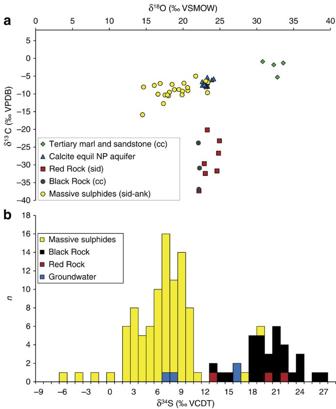Figure 3: Stable isotope geochemistry of the biogenic rocks at Las Cruces. (a) Carbon–oxygen isotope composition of carbonates (sid, siderite; cc, calcite; ank, ankerite), overlying Tertiary sandstone and marl, and calculated δ18O-δ13C isotope composition of calcite in equilibrium with the local groundwaters (25 °C). Isotopic composition of the calcite in equilibrium with the water has been calculated from the tabulated δ18O-δ13C values together with the fractionation factors of Kim and O’Neil45for oxygen and those of Romaneket al.46for DIC. For comparison, data are shown for the Variscan (primary-ore related) hydrothermal siderite–ankerite assemblage occurring in VMS deposits of the Iberian Pyrite Belt. (b) Sulphur isotope composition compared with the δ34Ssulphatevalues of the local groundwater and δ34S values of the primary sulphides at Las Cruces19. Figure 3: Stable isotope geochemistry of the biogenic rocks at Las Cruces. ( a ) Carbon–oxygen isotope composition of carbonates (sid, siderite; cc, calcite; ank, ankerite), overlying Tertiary sandstone and marl, and calculated δ 18 O-δ 13 C isotope composition of calcite in equilibrium with the local groundwaters (25 °C). Isotopic composition of the calcite in equilibrium with the water has been calculated from the tabulated δ 18 O-δ 13 C values together with the fractionation factors of Kim and O’Neil [45] for oxygen and those of Romanek et al. [46] for DIC. For comparison, data are shown for the Variscan (primary-ore related) hydrothermal siderite–ankerite assemblage occurring in VMS deposits of the Iberian Pyrite Belt. ( b ) Sulphur isotope composition compared with the δ 34 S sulphate values of the local groundwater and δ 34 S values of the primary sulphides at Las Cruces [19] . 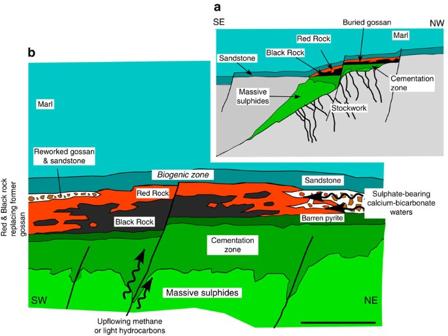Figure 4: Proposed model for the genesis of the biogenic carbonate–sulphide rocks of the Las Cruces deposit. (a) General idealized crosssection of the deposit. The SE–NW distance is ~300 m. (b) Cartoon based on the section depicted inashowing the proposed genetic model for the deposit. Carbonate–sulphide rocks (Red and Black rocks) formed in the supergene alteration zone (gossan) capping an older massive sulphide deposit. The porous gossan accumulated methane or light hydrocarbons that acted as electron donors for microbial reduction of aqueous sulphate transported by groundwater. This process destabilized goethite/haematite and oxidized minerals (beudantite, cerussite), leading to the formation of siderite, calcite, galena and silver-bearing sulphides, together with coarse-grained gold that has almost completely replaced the former gossan. Scale bar, ~50 m. Full size image Figure 4: Proposed model for the genesis of the biogenic carbonate–sulphide rocks of the Las Cruces deposit. ( a ) General idealized crosssection of the deposit. The SE–NW distance is ~300 m. ( b ) Cartoon based on the section depicted in a showing the proposed genetic model for the deposit. Carbonate–sulphide rocks (Red and Black rocks) formed in the supergene alteration zone (gossan) capping an older massive sulphide deposit. The porous gossan accumulated methane or light hydrocarbons that acted as electron donors for microbial reduction of aqueous sulphate transported by groundwater. This process destabilized goethite/haematite and oxidized minerals (beudantite, cerussite), leading to the formation of siderite, calcite, galena and silver-bearing sulphides, together with coarse-grained gold that has almost completely replaced the former gossan. Scale bar, ~50 m. Full size image Interpretation of the δ 34 S values for the sulphides is not straightforward, because the measured δ 34 S values are strikingly high compared with δ 34 S sulphate values of the groundwaters currently flowing into the open pit of the Las Cruces mine (+6.3 to +15.2‰) and with those of the underlying massive sulphides (−6.8 to +8.2‰) [8] , [19] ( Fig. 3b and Table 1 ). However, these high δ 34 S values are similar to those of associated barite (+20.4‰) [5] . This situation is rather unusual for biogenically mediated, sulphide-rich ore systems [20] , because strongly negative δ 34 S values are generally regarded as prima facie evidence of biogenic sulphate reduction [21] , [22] , whereas small Δ SO4-H2S values are characteristic of thermochemical sulphate reduction [23] . At the low temperatures expected in the secondary environment of the Las Cruces deposit (≈<70–80 °C), sulphate reduction can only be mediated biogenically, typically by dissimilatory anaerobic processes, whereas abiotic sulphate reduction is kinetically inhibited [23] . Some bacteria are known to excrete reduced sulphur with small Δ SO4-H2S values [24] . However, we interpret the isotopically high δ 34 S values as recording fractionation in a system having excess organic matter (TOC>>SO 4 2− ) and high rates of reduction, whereby all of the sulphate was rapidly transformed into sulphide [24] , [25] . The isotope values reflect the complete consumption of sulphate during anaerobic oxidation of electron donors in a closed system [26] , a process that is consistent with the high δ 34 S values of the sulphides. The presence of iron monosulphides is indicative of a low-fS 2 system and a limited availability of reduced sulphur. The ultimate origin of the groundwater sulphate is unknown, but it could have a seawater origin [27] , derived either from recent seawater intruding deep aquifers in the basin and upwelling along faults, or from the dissolution of accessory sulphate interbedded with the marl. The mineral assemblages of siderite–calcite and sulphides are unstable under sub-aerial oxic conditions, and in the Las Cruces deposit could only have formed in an aqueous environment enriched in CO 2 and, to some extent, in H 2 S. Thus, fluid–rock interactions should be able to produce three superimposed processes to form the observed assemblages: an increase of fCO 2 with stabilization of carbonates; a redox change with reduction of Fe 3+ to Fe 2+ , also related to the replacement of goethite/haematite by siderite; and sulphidization accompanied by the deposition of the sulphides. The evolution of the gossan to the Red Rock must involve a complex set of reactions summarized as follows: Microbes facilitating the classical reaction with methane and sulphate, producing CO 2 and H 2 S (reaction 1), should be associated with another consortium of anaerobic bacteria that, in the presence of excess goethite, favour reaction (2) in which the goethite acts as an electron acceptor; this reaction is favoured due to its low free energy of formation [28] . Reactions (1) and (2) involve the oxidation of an electron donor, here represented by methane, but could well be organic molecules having low molecular weight. The low δ 13 C values exclude hydrogen as the main electron donor and point instead to the involvement of methane or light hydrocarbons. The reduction of Fe 3+ to Fe 2+ associated with the replacement of goethite by siderite (reactions 2 and 3) is also probably due to bacterial activity. In surficial low-temperature environments, the reduction of Fe 3+ to Fe 2+ occurs predominantly by biogenic processes [29] , [30] . Abiogenic reduction of iron is unlikely to take place at Las Cruces because in surficial settings it has only been observed to occur in relationship with photoreduction [31] and in some immature, organic matter-rich environments such as soils. In the latter setting, abiogenic reduction is associated with the oxidation of quinone-rich humic acids and phenolic compounds [32] , derived mainly from plant tissues. Even in the presence of organic compounds capable of reducing Fe 3+ , the extent of abiotic iron reduction is much less than that produced by biological reduction [28] and, moreover, the actual role of phenolic compounds in direct abiotic reduction, or as electron shuttles from bacteria to Fe 3+ mineral surfaces, is controversial. The H 2 S generated during reaction (1) should increase fS 2 , leading to the destabilization of the cerussite and precipitation of galena Finally, the formation of the Black Rock is related to replacement of the siderite by calcite: In a strict sense, reactions (1) and (2) are not needed for the stabilization of the carbonate, because the flowing groundwater carries CO 2 and, hence, reaction (1) could be replaced by However, again the carbon isotope signatures indicate a significant input of carbon derived from the bacterial metabolization of methane/organic matter, therefore suggesting that reactions (1) and (2) are indeed relevant. The precipitation of pyrite seems to be kinetically inhibited in the Black Rock. Instead, amorphous or poorly ordered greigite or smythite have precipitated. Although these minerals have been formed abiotically in the laboratory [33] , [34] , Kucha and Barnes [35] and Raiswell and Plant [36] proposed that the presence of such intermediate-valence monosulphides is directly related to biogenic precipitation. At Las Cruces, crystallization of these iron sulphides inhibited the formation of siderite and rendered calcite the stable carbonate in the presence of high aCa 2+ /aH +2 . There is no available Ca 2+ in the replaced gossan and, thus, we infer it is derived from the calcium-bearing groundwaters. Formation of the complex Ag-As-Fe-Cu sulphosalts intergrown with the galena is interpreted as being related to destabilization of the Ag-bearing jarosite and to input of sulphur of biogenic derivation. We also interpret the formation of free gold as being linked to bacterial activity: during sulphidization of the gossan, sub-microscopic ‘invisible’ gold [11] was transformed into coarse grains; by analogy, multiple lines of evidences have been presented for the biogenic formation of gold nuggets [37] , [38] . Dissimilatory sulphate-reducing microbes have played a key role in the formation of many low-temperature stratiform ore deposits, with the reduced sulphur being derived from extensive biogenic reduction of dissolved sulphate [22] , [39] , [40] . Other sub-surface microbial activity is related to the secondary alteration of sulphides into oxides and carbonates [41] . During this supergene alteration, lithoautotrophic bacteria accelerate the dissolution of exposed ore deposits and promote the precipitation of secondary sulphides within the cementation zone, accelerating the process by up to five orders of magnitude above abiotic processes [42] , [43] . Biogenically mediated supergene precipitation of other sulphides has been described elsewhere, such as in the present-day formation of sphalerite biofilms in the Mike gold mine, in Nevada, USA [23] . We propose that the unusual mineral assemblage found in the secondary zone of the Las Cruces ore deposit formed in a large natural bioreactor, where coupled microbial sulphate reduction and methane oxidation took place below a thick impermeable marl unit. The preferred site for such biogenic activity is where sulphate-bearing groundwaters interacted with a previously formed porous gossan, which was also the zone of gas accumulation beneath the sealing marl ( Fig. 4 ). Under these conditions, anaerobic sulphate-reducing microbes were able to reduce the aqueous sulphate that then reacted in situ with the available metals; in fact, the metal assemblage found within this biotic zone is the same as that found in the gossans of the Iberian Pyrite Belt [11] . This process would be synchronous with the release of CO 2 as a byproduct of the heterotrophic metabolism of anaerobic microbes; mixing of this carbon with DIC transported by the groundwater produced supersaturation in, and precipitation of, carbonates. The inferred high CH 4 /SO 4 ratios should promote quick and nearly complete sulphate reduction and the anomalously high sulphur isotope signatures. An estimation of the tonnages and metal grades of the Red and Black rocks, based on mineral compositions and abundances, suggests that the sub-surface microbial system at Las Cruces has modified the mineralogy of at least 2–6 km 3 of rock, fixing at least 1.09 × 10 10 moles of CO 2 and 3.1 × 10 9 moles of H 2 S, and resulting in the formation of ca . 1.19 Mt of siderite and calcite, 114,000 t of galena, 638 t of silver sulphides and 6.5 t of free gold ( Table 2 ). Such quantities reflect the existence of a vast underground microbial system, with the limiting factor in this system probably being the availability of electron acceptors. Table 2 Calculation of the amounts of sulphides produced by biogenic activity at Las Cruces. Full size table The exact timing of the ore-forming process is difficult to constrain, because the assemblage lacks minerals suitable for accurate absolute dating. Geological relations suggest that the main gossan formation took place at 8–7 Ma (ref. 11 ) and that this gossan was covered by sediments at ca . 7.2–5.3 Ma; crosscutting relationships indicate that the deposition of galena postdated the formation of the underlying cementation zone and the overlying marl. Hence, the ore-forming event took place between burial at 7.2–5.3 Ma and the present. However, the microbially mediated mineralizing system has not changed significantly since burial and, thus, it may still be an active process. Our model for the formation of secondary Pb-Ag-Fe sulphides and gold is different from those invoked for all known biogenically mediated ore-bearing systems. Equivalent secondary mineral assemblages are virtually unknown in the Earth’s crust; the only broadly comparable assemblages that have been reported are in the small Zapadno–Ozernoe mine, in the Russian Urals [44] . The formation of the large bioreactor in the subsurface at the Las Cruces deposit probably involves a wide community of competing chemolithotrophic microbes resulting in mineral-forming processes that are influenced and controlled by fluctuations in water input, temperature and availability of nutrients. Variations in any of these limiting factors and the nature of the aerobic/anaerobic interface probably control the size and resulting mineralogy of this vast underground ecosystem. Sampling and preparation Selected samples of ore, overlying sediments and waters were collected in situ from outcrops in the open pit; 1–3 g of individual minerals (carbonates and galena) were selected under the binocular microscope or separated magnetically (iron monosulphides); in the cases of finely intergrown assemblages, the gases were separated chemically following the procedures described below. Isotope measurements Carbon dioxide was obtained by reaction of the carbonates [47] , [48] and DIC [49] with 100% phosphoric acid. Water was analysed using the CO 2 –H 2 O equilibration method of Epstein and Mayeda [50] . For analysis of δD, an aliquot of water (0.5 μl) was injected into a ceramic column containing a glassy carbon tube at 1,400 °C to produce H 2 and CO gases [51] . Sulphur isotopes of dissolved sulphates were measured after precipitation of BaSO 4 from solution. SO 2 was obtained from the barium sulphate as well as from the sulphides by combustion with V 2 O 5 and O 2 at 1,030 °C (ref. 52 ). Isotope measurements were carried out at the Stable Isotope Laboratory of the Instituto Andaluz de Ciencias de la Tierra (CSIC-UGR, Granada) with a Delta Plus XL (ThermoQuest, Bremen, Germany) mass spectrometer (elemental analysis–isotope ratio mass spectrometry) for sulphur, oxygen in sulphate, and water and deuterium isotope analyses, and a Delta Plus XP spectrometer for C and O isotopes in carbonates. Precision was calculated, after correction of the mass spectrometer daily drift, from data obtained on standards systematically interspersed in analytical batches, at better than ±0.1‰ for δ 13 C for carbonates and DIC, and for δ 18 O carbonates and water oxygen. Precision was better than ±0.2‰ for sulphate sulphur (δ 34 S) and for sulphate oxygen (δ 18 O), and better than ±2‰ for water hydrogen (δδD). The standard for reporting carbon measurements is VPDB (Vienna-PDB), for oxygen and hydrogen is VSMOW (Vienna Standard Mean Oceanic Water) and for sulphur is VCDT (Vienna Canyon Diablo Troilite). Scanning electron microscope/energy-dispersive spectrometer analyses Small, ca 2.5-mm grains of the Black Rock were analysed under a Jeol 5600-LV scanning electron microscope equipped with an Oxford Industries INCA X-sight energy-dispersive spectrometer at the Centro de Astrobiología. Backscattered and secondary electron images and energy-dispersive spectra were obtained on samples mounted on Al stubs and without coating ( V =20 kV; I =85 μA, electron beam diameter=1 μm). Quantitative analysis performed on several (21) bacteriomorphic structures show that they are made of galena (mean 84.89±1.49% wt Pb, 15.11±1.02% wt S) with only negligible traces of other elements present. How to cite this article : Tornos, F. et al. Formation of recent Pb-Ag-Au mineralization by potential sub-surface microbial activity. Nat. Commun. 5:4600 doi: 10.1038/ncomms5600 (2014).